Bending rules for animal propulsion Animal propulsors such as wings and fins bend during motion and these bending patterns are believed to contribute to the high efficiency of animal movements compared with those of man-made designs. However, efforts to implement flexible designs have been met with contradictory performance results. Consequently, there is no clear understanding of the role played by propulsor flexibility or, more fundamentally, how flexible propulsors should be designed for optimal performance. Here we demonstrate that during steady-state motion by a wide range of animals, from fruit flies to humpback whales, operating in either air or water, natural propulsors bend in similar ways within a highly predictable range of characteristic motions. By providing empirical design criteria derived from natural propulsors that have convergently arrived at a limited design space, these results provide a new framework from which to understand and design flexible propulsors. Thrust production by propulsive structures is a fundamental requirement for animal movement through air or water. Models of animal propulsion often emulate patterns that have been established for hydrofoils and airfoils [1] , [2] , [3] , [4] , [5] and, as with these engineering-based models, animal propulsor models often assume a rigid structure that oscillates through the surrounding fluid with varying types of heaving and pitching motions [6] , [7] . However, animal propulsors are not rigid, but instead, typically bend during motion ( Fig. 1 ). Attempts to evaluate the role of propulsor bending on thrust production have been met with conflicting results. For example, although some empirical [8] , [9] , [10] , modelling [11] , [12] , [13] and computational studies [14] , [15] , [16] , [17] have indicated that flexible propulsors may permit higher thrust production than rigid counterparts, other evidence indicates that flexibility may sometimes lessen or prevent thrust production [10] , [18] , [19] . Evaluation of these results has been complicated by a lack of common bending criteria to guide experimental design. Consequently, bending has been projected to occur both evenly over the full length [17] , [20] and only over a limited portion [21] , [22] of the propulsor. Most frequently, flexibility has been evaluated in terms of material properties such as elastic modulus [10] , [17] or flexural stiffness [19] , [23] , [24] of the propulsor rather than actual bending patterns. Experimental testing of the effects of bending on thrust production have been influenced by the inherent control possible with human-engineered propulsors so that most work on flexibility has been based on specifically engineered propulsors in laboratory conditions. Rarely have bending patterns of living animal propulsors, which have evolved over millions of years and among multiple taxonomic groups, been measured to inform experimental manipulations. 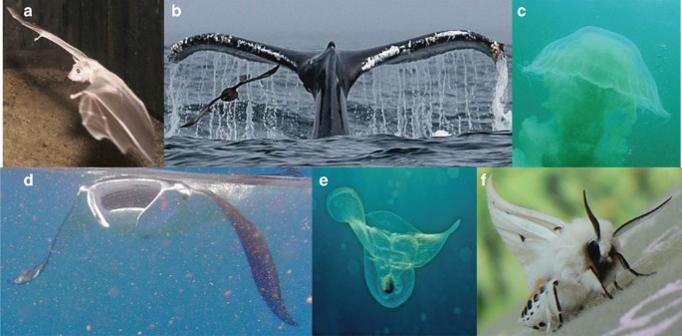Figure 1: Diversity of flexible tips among natural propulsors. A wide array of distantly related animal groups employ flexible margins on their propulsive structures, including (a) the wings of bats, (b) flukes of cetaceans such as humpback whales and wings of sea birds (in foreground), (c) the bell margin of large rowing scyphomedusae, (d) the fins of fish such as manta rays, (e) the wing-like foot of pteropod molluscs and (f) the wings of a variety of insects such as large moths (image sources listed in acknowledgement section). Images illustrate propulsor bending but may not represent conditions of steady propulsion. Figure 1: Diversity of flexible tips among natural propulsors. A wide array of distantly related animal groups employ flexible margins on their propulsive structures, including ( a ) the wings of bats, ( b ) flukes of cetaceans such as humpback whales and wings of sea birds (in foreground), ( c ) the bell margin of large rowing scyphomedusae, ( d ) the fins of fish such as manta rays, ( e ) the wing-like foot of pteropod molluscs and ( f ) the wings of a variety of insects such as large moths (image sources listed in acknowledgement section). Images illustrate propulsor bending but may not represent conditions of steady propulsion. Full size image Here we describe, based on measurements of bending patterns across diverse animal taxa, universal patterns of animal propulsor bending, which transcend differences in fluid medium, animal size or phylogenetic background. Patterns of propulsor tip bending Comparison of video sequences (see Supplementary Data 1 and 2 ) for 59 animal species demonstrates clear, replicable patterns of spanwise propulsor bending during steady motion, which are similar over a broad range of animal sizes, fluid media and taxonomic groups. The position of propulsor bending is documented as the flexion ratio (length from propulsor base to flexion point of bending relative to the total propulsor length). In addition, the maximum extent of propulsor bending is measured as the maximum flexion angle (referred to simply as flexion angle). Both flexion ratio and angle vary significantly between individual species (analysis of variance (ANOVA), n =59, df=58, F=6.7 for ratio, 8.8 for angle, P <0.001 for both variables) but only within constrained ranges for both flexion ratio and flexion angle ( Fig. 2 ). The two variables form a discrete set of combinations ( Fig. 3 ), or morphospace [25] , [26] , [27] , within the range of potentially available combinations. Although the ranges of both variables are strongly limited, there is no significant linear relationship between the two measures of propulsor bending (simple linear regression, N =59, df=1, 57, P =0.46, r 2 =0.009), indicating that each variable may be selected independently. The relative consistency of these two bending measures across such a wide array of animal propulsors suggests strong conservation of bending geometry during steady motion among animal taxa operating within inertially dominated fluid flows. 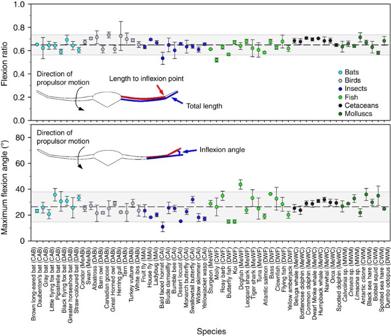Figure 2: Patterns of propulsor bending by a variety of animals moving steadily through air and water. (Top) The position of bending, or flexion ratio and (Bottom) average maximum flexion angle during bending. Diagrams inset within each panel illustrate the flexion measure for an orthogonally viewed animal (examples of the measurements for each animal group are illustrated inFig. 5). The species depicted are listed along the bottom axis by common name (source video locations inSupplementary Data 1, species name and additional data inSupplementary Data 2). The categorical codes accompanying animal names refer to animal’s approximate overall body length (M, millimetre (0.001–0.01 m); C, centimetre (0.01–0.1 m); D, decimetre (0.1–1.0 m); Me, metre (.1.0 m)), fluid medium (A, air; W, water) and taxonomic group (B, bats; Bi, birds; I, insects; F, fish; C, cetaceans; M, molluscs). Data points represent average values (N=the number of individuals for each species, seeSupplementary Data 2) of individual species and error bars indicate±one s.d. from the species mean. Dashed lines represent mean values and shaded regions the 95% confidence intervals for all species combined (N=59, flexion ratio mean=0.65, 95% interval=0.56–0.74; flexion angle mean=26.5, 95% interval=14.5–38.4). All points represent conditions of steady propulsion through inertially dominated fluid flows. Figure 2: Patterns of propulsor bending by a variety of animals moving steadily through air and water. (Top) The position of bending, or flexion ratio and (Bottom) average maximum flexion angle during bending. Diagrams inset within each panel illustrate the flexion measure for an orthogonally viewed animal (examples of the measurements for each animal group are illustrated in Fig. 5 ). The species depicted are listed along the bottom axis by common name (source video locations in Supplementary Data 1 , species name and additional data in Supplementary Data 2 ). The categorical codes accompanying animal names refer to animal’s approximate overall body length (M, millimetre (0.001–0.01 m); C, centimetre (0.01–0.1 m); D, decimetre (0.1–1.0 m); Me, metre (.1.0 m)), fluid medium (A, air; W, water) and taxonomic group (B, bats; Bi, birds; I, insects; F, fish; C, cetaceans; M, molluscs). Data points represent average values ( N =the number of individuals for each species, see Supplementary Data 2 ) of individual species and error bars indicate±one s.d. from the species mean. Dashed lines represent mean values and shaded regions the 95% confidence intervals for all species combined ( N =59, flexion ratio mean=0.65, 95% interval=0.56–0.74; flexion angle mean=26.5, 95% interval=14.5–38.4). All points represent conditions of steady propulsion through inertially dominated fluid flows. 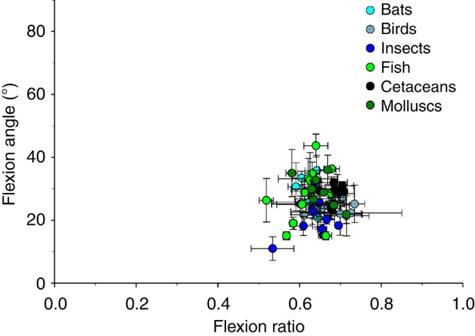Figure 3: Flexion morphospace of natural propulsors during steady motion. Axes encompass a potential range of flexion distributions and the data points represent the empirically observed subset of the potential space. Data points are means for each species (N=number of individuals of each species, seeSupplementary Data 2), and error bars indicate±one s.d. from the species mean for both flexion ratio and angle. The relationship between flexion ratio and angle is not linear (simple linear regression,N(number of species)=59, df=1, 57,P=0.46,r2=0.009). Full size image Figure 3: Flexion morphospace of natural propulsors during steady motion. Axes encompass a potential range of flexion distributions and the data points represent the empirically observed subset of the potential space. Data points are means for each species ( N =number of individuals of each species, see Supplementary Data 2 ), and error bars indicate±one s.d. from the species mean for both flexion ratio and angle. The relationship between flexion ratio and angle is not linear (simple linear regression, N (number of species)=59, df=1, 57, P =0.46, r 2 =0.009). Full size image Statistical analysis integrating phylogenetic signal Individual species (two to four individuals of each species, see Supplementary Data 2 ) were comparatively robust for their propulsor flexion traits. Replicate cycles of propulsor motion for particular individuals (2–15 cycles for each individual of a species) do not contribute significantly to variance of either flexion ratio (ANOVA, n =557, df=11, P =0.99) or angle (ANOVA, n =574, df=14, P =0.28). When replicates for each individual are grouped, individuals of a species do not contribute significantly to variations in flexion ratio (ANOVA, n =157, df=3, P =0.38) or angle (ANOVA, n =157, df=3, P =0.51). Central tendencies of the flexion variables are relatively insensitive to small (<30%) errors introduced into the data set by the generation of random errors within the measurements ( Supplementary Fig. 1 ). Owing to the low variation found between propulsive cycles of a single individual and between individuals of the same species, values for individuals of the same species were combined and analysis focused on variations in bending patterns between species. The distributions of interspecific flexion variables were generally normal within species categories (size, fluid medium and taxonomic groupings). With one exception (flexion angle for the group of animals a metre or more in length), the distributions of flexion ratio and angle values for species categories did not deviate significantly from normal distributions ( Supplementary Table 1 ). Similarly, variances within species categories did not deviate significantly from homogeneity ( Supplementary Table 2 ). The similarity in flexion ratio and angle distributions within species categories therefore satisfied the essential assumptions for comparison between the categories using ANOVA methods. We considered the potential role of phylogenetic signal in bending patterns among animal groups because phylogenetic relationships may contribute to pattern formation for a range of variables among related taxa. Most broadly, phylogenetic signal is the tendency for evolutionarily related organisms to resemble each other without identification of the mechanism that might cause such resemblances. Phylogenetic signal has been detected at significant levels in comparative studies of animal traits, particularly when more than 20 species are compared [28] and consequently might be expected within the flexion data. This would have an impact on our analysis if similarities of bending patterns between animal groups are confounded by phylogenetic relatedness between groups. In this case, rather than each species representing a separate and independent set of observations, species that were phylogenetically closer might be expected to have more similar patterns and would not be statistically independent, as assumed during statistical hypothesis testing. Blomberg’s [28] K values above 1.0 demonstrate strong phylogenetic relatedness for the variable considered whereas values below 1.0 indicate that species resemble each other less than expected based solely on a Brownian motion model of trait evolution along the phylogenetic tree. Phylogenetic signal was relatively low (<1.0) but significantly present within the data for both flexion variables (flexion ratio: K =0.56, P =0.004; flexion angle: K =0.67, P <0.001, Supplementary Table 3 ). The presence of significant phylogenetic signal within the flexion data necessitated a statistical approach (phylogenetic ANOVA [29] ) that incorporates this information. 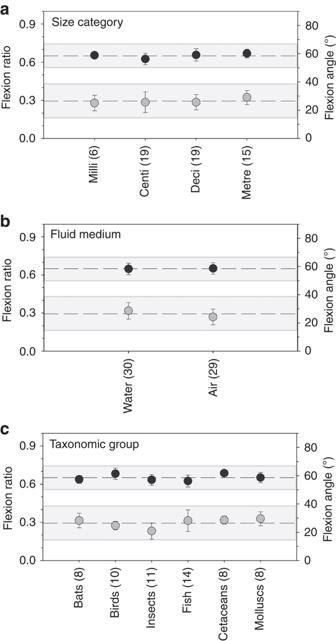Figure 4: Generality of bending patterns across a variety of animal categories. Data points represent mean values±one s.d. for each of the groups (a-size,b-fluid,c-taxon) listed along the bottom axis. Species were grouped according to criteria listed inFig. 2and parenthetical numbers represent the number of species (N) comprising a listed group. Dashed lines and shaded regions represent the same mean and 95% confidence intervals as inFig. 2. Where not visible, s.d. lines are encompassed within the data point symbol. Phylogenetic ANOVA indicated that differences in flexion traits between categorical variables (size class, fluid medium and taxonomic group) were not significant when considering the phylogenetic signal within the data (all P >0.1, Supplementary Table 4 ). Graphic analysis of means and confidence intervals ( Fig. 4 ), illustrated differences in flexion variables that would be considered small, but significant, using a conventional one-way ANOVA approach. However, inclusion of genetic distance information ( Supplementary Fig. 2 , Supplementary Data 3 ) within a phylogenetic ANOVA demonstrated that when the genetic relatedness of the species within the data was considered, the differences between major categorical variations were not significant ( Supplementary Table 4 ). Figure 4: Generality of bending patterns across a variety of animal categories. Data points represent mean values±one s.d. for each of the groups ( a -size, b -fluid, c -taxon) listed along the bottom axis. Species were grouped according to criteria listed in Fig. 2 and parenthetical numbers represent the number of species ( N ) comprising a listed group. Dashed lines and shaded regions represent the same mean and 95% confidence intervals as in Fig. 2 . Where not visible, s.d. lines are encompassed within the data point symbol. Full size image We include a conventional ANOVA analysis that does not consider genetic distances because, although the phylogenetic ANOVA is the appropriate hypothesis testing method for a situation involving significant phylogenetic signal, comparison of phylogenetic and conventional ANOVA approaches provides insight into patterns within the data. Graphical evaluation using 95% confidence intervals demonstrated a very limited morphospace for both flexion variables ( Figs 2 , 3 , 4 ) and the phylogenetic ANOVA demonstrates that the minor variations between grouping variables can be explained by phylogenetic proximity of the taxa being compared rather than some important influence of size, medium or structural differences between the taxa. However, the utility of the conventional ANOVA lies with its implication that, within the constrained design space for propulsor flexion, small absolute differences are most likely to be found among groups with comparatively large phylogenetic distances. For example, propulsor flexion angle is, on average, lower for insects than for several other animal taxa ( Fig. 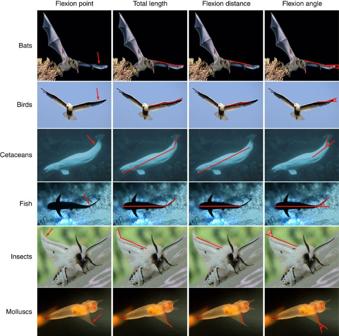Figure 5: Illustration of the flexion measurements for each major taxonomic group considered in the flexion data set. Columns represent the variable measured and rows contain a representative image for each major taxonomic group considered. 4c , Supplementary Table 5 ). Insects are a comparatively basal group among those we considered ( Supplementary Fig. 2 ). Similarly, within the vertebrates, fish are more likely to have lower flexion ratios than other taxa ( Fig. 4c , Supplementary Table 5 ). The differences indicated by the conventional ANOVA do not result in large variations within the overall design spaces of the flexion variables ( Fig. 4c ) but reflect the phylogenetic distances over which these lineages have evolved during convergence on a restricted design space for propulsor bending. The remarkable consistency of animal bending patterns across animal sizes, fluid media or taxonomic groups leads to some unexpected results. For example, it is not coincidental that, during steady motion, the wings of an airborne monarch butterfly bend in a proportionately similar location and to a similar maximum angle as the tail of a swimming bottlenose dolphin or the wing-foot of the molluscan pteropod, Clione antarctica ( Fig. 2 ). These are examples of common bending patterns that remain consistent across groups with exoskeletons (insects), endoskeletons (birds, bats, fish and cetaceans) or hydrostatic skeletons (molluscs). The propulsors may be actuated (birds, bats, fish, cetaceans and molluscs) or completely passive (insects). The material compositions of these propulsors vary dramatically (for example, chitin, feathers and bones) among taxa. These data suggest that, rather than being determined by structural designs or material compositions, bending patterns of animal propulsors are constrained to a relatively narrow range of kinematic criteria. In turn, this suggests a key distinction between material properties (for example, elastic modulus, flexural stiffness, material resonance and joint patterns) and systems requirements (bending kinematics) of animal propulsors. Material properties are necessary conditions for flexible propulsors, but the universality of animal bending patterns demonstrates that the necessary material and structural requirements for propulsor bending have been resolved in many ways by many different animal taxa. Most importantly, the universality of the bending patterns demonstrates that a limited set of system requirements, primarily bending kinematics, are fundamentally important for flexible biological propulsion. What factor(s) drive natural selection to converge on highly constrained bending kinematics across such a wide range of animal groups? Energetic efficiency of thrust production probably provides both advantages and constraints on bending designs. Propulsor margin bending can increase vortex circulation and generate pressure gradients [22] around propulsors, which results in thrust enhancement of a factor >10 2 relative to rigid propulsors [21] . The energy savings accrued through maximizing energetic efficiency during thrust production may strongly favour evolutionary convergence on designs that produce such thrust advantages. Vortex circulation, thrust production and efficiency vary with flexibility, suggesting that the flexibility of animal propulsors may be tuned to maximize thrust production and efficiency [30] , [31] , [32] , [33] by controlling vorticity associated with propulsor bending. For example, although some bending is favourable, extensive bending can lessen thrust production efficiency [18] by disrupting vortex organization along the span of a propulsor [10] . Similarly, specific spatial and temporal alignments of adjacent opposite-spin vortices at the tips of propulsor margins are crucial for production of fluid jets produced at vortex interfaces [34] , [35] . As propulsor geometries and kinematics control spatial and temporal distributions of vorticity [36] , [37] , propulsor geometries and kinematics are key determinants of thrust production in fluids. Even subtle bending kinematics influence alignment of vortices, which determine the energetic efficiency of propulsion [38] , and may be subject to strong natural selection. Small variations in bending patterns among taxonomic groups resemble model predictions that weak, but significant, phylogenetic signal may reflect strong stabilizing selection within constrained boundaries acting on phylogenetically disparate species groups [39] . The bending pattern morphospace demonstrates a degree of design latitude, but the generally narrow range of natural propulsor flexion patterns indicates strong selection during the evolution of animal propulsors towards a tightly constrained range of bending kinematics. The wide diversity of propulsor material and actuation traits following these design rules demonstrate that a diversity of properties have been modified by different animal taxa operating in different fluids to reach similar geometric arrangements of propulsor bending. The narrow range of observed natural propulsor geometries parallels other documented kinematic patterns of natural propulsors. Steady propulsion has been found to conform to a Strouhal number (St= fA / U , where ( f ) stroke frequency and ( A ) amplitude are divided by ( U ) forward speed) range of ~0.2–0.4 for animals moving within inertially dominated fluid flows [40] . Like propulsor bending patterns, St conservation occurs uniformly across wide animal length scales, fluid media and taxonomic groups [40] , [41] . Also, similar to propulsor bending patterns, St conservation is believed to permit efficient generation and control of vortices, which results in maximum thrust efficiency per propulsor energy input [42] , [43] . Constrained propulsor bending and Strouhal number conservation may be related. However, further exploration of the specific fluid interactions underlying these universal patterns is necessary to clarify our understanding of animal propulsion and provide essential design rules for creating successful biomimetic propulsors. Human-engineered propulsors may then benefit from patterns developed over millions of years of evolutionary selection within the animal kingdom. Data sources and quantification of propulsor flexion Video sequences of animals ( N =59 species) in steady-state swimming or flight were collected from various online sources (for example, YouTube, Vimeo and so on) using YouTube Downloader freeware (DVDVideoSoft). Internet addresses from which videos were accessed are given in Supplementary Data 1 and the complete data set, including all replicate sample values, is given in Supplementary Data 2 . Animals were selected based on their use of oscillatory motions of their propulsors. Animals with highly undulatory motions such as eels and animals augmenting their forward motion with other appendages (such as the walking limbs of a reptile) were not considered. While there are several lineage-dependent patterns of propulsor bending associated with internal body structure (for example, joint structures of birds, bats, fish and mammals), our goal was to characterize bends solely due to propulsor flexibility, so we used the flexion point of the bend closest to the propulsor tip for all animal lineages. The selected animals represented divergent taxa (bats, birds, insects, fish, cetaceans and molluscs), and the propulsors comprised many different materials (skin membrane, feathers, chitin, bone and so on). Animal size range included ~0.005 m Limacina helicina , a pteropod mollusc (Re~40), up to ~8.4 m orca whale ( Orcinus orca ) (Re~10 7 ). Animals were selected based on availability of video, such that at least two (range 2–4) individuals of the same species were represented, with each of these individuals undergoing multiple (average 3, range 2–15) propulsive cycles ( Supplementary Data 2 ). Rapid acceleration events often included transient, extensive propulsor bending and were not included in the analysis. Instead, sequences were chosen to represent steady-state conditions in which propulsor motions were relatively even between consecutive propulsor movement cycles. Two variables were measured to characterize the kinematics of the propulsor margin: the location (flexion ratio) and the magnitude (flexion angle) of bending ( Fig. 2 ). These features were measured on video frames using the application ImageJ (NIH). Flexion angle was defined as the angle of the margin’s bend away from the central propulsor axis. To obtain this angle, the obtuse angle between the flexion point and distal propulsor tip was measured using ImageJ. This obtuse angle was the supplement of the acute flexion angle (illustrated with examples for each major taxonomic group in Fig. 5 ). The flexion ratio was defined as the length along the propulsor from the propulsor base to the flexion point relative to the total length of the propulsor. High flexion ratios (close to 1.0) indicated a flexion point located more distally along the propulsor ( Figs 2 and 5 ). Figure 5: Illustration of the flexion measurements for each major taxonomic group considered in the flexion data set. Columns represent the variable measured and rows contain a representative image for each major taxonomic group considered. Full size image Measurements throughout a particular propulsion cycle required conversion of video sequences into a series of images representing successive stages of propulsor motion using Adobe Premiere Pro CS3 software. Alternate frames were used for each image series, except where propulsor oscillations occurred so quickly that all frames were used to provide adequate resolution of motions. The flexion angle was measured on each still image extracted from a video sequence. As the magnitude of the flexion angle varied throughout the propulsive cycle, only the maximum amplitude of flexion angle in each cycle was considered during further analyses. Flexion ratio was measured multiple times per propulsive cycle (average 3.5, s.d. 1.4) and the maximum flexion angle was measured over multiple propulsive cycles (average 2.9 cycles, s.d. 2.2) for each replicate individual of a species. The full range of bending variation over a pulsation cycle was evaluated by taking measurements throughout pulsation cycles (average 9.9, s.d. 7.5 measurements per cycle). Propulsor tip bending occurred over a range of propulsor orientations relative to oncoming fluid flow. Therefore, both the streamwise tip bending of birds, bats, insects and molluscs, and the spanwise bending of fish and cetaceans were measured ( Fig. 5 ). Accurate measurement of the flexion angle optimally required an orthogonal view of the propulsor and this was a key criterion for video sequence selection. For fish, this meant that we used only views looking directly upwards or downwards on the fish. For close-up sequences of flying animals, only directly orthogonal views were used. With distant views, commonly used for birds, only sequences in which the bird was flying towards or away from the camera were selected. The flexion data set does not have completely parallel flexion ratio and angle data—not all video sequences had identical numbers of replicates. This is because image sequences were not always suitable for collection of both types of data in the same scene. Consequently, sample sizes for each species were not uniform ( Supplementary Data 2 ). Owing to the diverse sources of videos used for flexion measurements, we evaluated the sensitivity of flexion measurements to measurement variations such as might accompany deviations from orthogonality. Random corruption of the original flexion data demonstrated that central tendencies of the flexion variables were relatively robust. Although variance around mean values increased, average values for flexion ration and angle remained stable when random errors of 10, 20 and 30% were introduced into the original data set ( Supplementary Fig. 1 ). This pattern indicates that small (<30%) errors introduced into the data set during variable measurements or by minor deviations from orthogonality of images would be unlikely to alter central patterns within the data set. Phylogenetic signal evaluation A phylogenetic hypothesis of relationships among taxa and species used for propulsor flexion analysis was generated based on mitochondrial cytochrome c genetic data available through GenBank ( Supplementary Data 3 ) using MEGA [44] . The resulting phylogenetic tree ( Supplementary Fig. 2 ) was consistent with contemporary phylogenetic hypotheses describing animal evolution [45] , [46] . Phylogenetic distances from that tree were then used to calculate Blomberg’s K and its level of significance [28] for both experimental variables. The presence of significant phylogenetic signal influenced the choice of ANOVA used to compare flexion variables between animal groups. Significant phylogenetic signal within flexion traits ( Supplementary Table 3 ) indicated that average values for phenotypes did not represent independent or random data points. This is true within a restricted lineage as well as within a larger grouping involving multiple animal lineages. Consequently, degrees of freedom may be inflated and significance levels derived from conventional tests may become unreliable when there is significant phylogenetic signal present [28] . However, phylogenetic signal can be included within ANOVA procedures to permit comparative analyses that account for evolutionary relatedness of traits among clades. Consequently, we used a phylogenetic ANOVA [29] to analyse patterns of flexion kinematics among animal groups. How to cite this article: Lucas, K. N. et al. Bending rules for animal propulsion. Nat. Commun. 5:3293 doi: 10.1038/ncomms4293 (2014).